Spin readout and addressability of phosphorus-donor clusters in silicon The spin states of an electron bound to a single phosphorus donor in silicon show remarkably long coherence and relaxation times, which makes them promising building blocks for the realization of a solid-state quantum computer. Here we demonstrate, by high-fidelity (93%) electrical spin readout, that a long relaxation time T 1 of about 2 s, at B =1.2 T and T ≈100 mK, is also characteristic of electronic spin states associated with a cluster of few phosphorus donors, suggesting their suitability as hosts for spin qubits. Owing to the difference in the hyperfine coupling, electronic spin transitions of such clusters can be sufficiently distinct from those of a single phosphorus donor. Our atomistic tight-binding calculations reveal that when neighbouring qubits are hosted by a single phosphorus atom and a cluster of two phosphorus donors, the difference in their electron spin resonance frequencies allows qubit rotations with error rates ≈10 −4 . These results provide a new approach to achieving individual qubit addressability. Silicon is an attractive material to host spin qubits because of its low spin–orbit coupling and natural abundance of zero nuclear spin isotopes, leading to long decoherence ( T 2 ) (refs 1 , 2 , 3 ) and relaxation times ( T 1 ) (refs 4 , 5 , 6 ). Particularly, in bulk P-doped Si (Si:P), a remarkably long T 1 was measured (≈3,000 s at T =1.3 K and B =320 mT) in ref. 4 . Recent results have demonstrated high-fidelity electron spin readout of a single implanted P donor in silicon with T 1 =6 s at T =100 mK and B =1.5 T (ref. 6 ), thereby establishing one of the key milestones of realizing a scalable spin quantum computing architecture [7] , [8] , [9] . Here, we demonstrate that long T 1 is retained also for electronic spin states bound to an ultra-small cluster of P donors, precisely engineered by scanning tunnelling microscope (STM) hydrogen lithography. STM-patterned device layout The spin readout architecture used in this study consists of an ultra-small donor cluster (≈4 P donors), both tunnel and capacitively coupled to an adjacent single electron transistor (SET) ( Fig. 1a ). Exploiting the atomic-scale precision of STM hydrogen lithography, this planar architecture was fabricated and previously demonstrated to exhibit high contrast charge-sensing characteristics [10] . To review the device layout, Fig. 1b shows a filled-state STM image, where the yellow features correspond to the device template, generated by desorbing the hydrogen resist monolayer (blue) with the STM tip. Subsequent exposure of the Si surface to PH 3 gas and annealing incorporate P donors, only within the device pattern [10] . A close-up of the central part of the device, after the lithography step, is seen in Fig. 1a . The two terminals source (S) and drain (D), along with the island D 1 , define the SET. The pattern which creates the P-donor cluster (D 2 in Fig. 1a ) is situated at a distance of 16 nm from D 1 . Two gates G 1 and G 2 are optimally situated ( Fig. 1b ) to gain sufficient differential control of the electrochemical potentials of D 1 and D 2 ( μ D1 and μ D2 ). 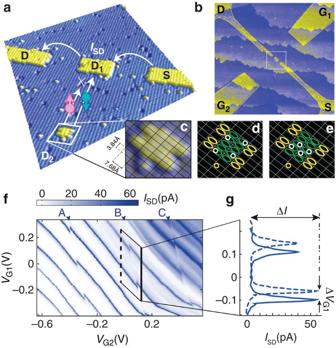Figure 1: Spin readout architecture for donor clusters. (a) Central part of the device (in yellow), patterned by desorbing the hydrogen mask (in blue), showing the SET island (D1), the few-donor quantum dot (D2), and the innermost sections of the source and the drain leads of the SET. Spin-dependent tunnelling between D1and D2is shown schematically. (b) The overall device, showing the layout of the two gates (G1, G2) and the extensions of the S and D leads. The white box shows the area shown ina. (c) Close-up image of D2, overlaid by a grid with dimer-row spacing, revealing the exposed silicon dimers. (d,e) Schematic representation of D2, showing sites suitable for P donor incorporation in green and the rest in yellow. The set of four white circles show two possible configurations of the P donors. (f) Map of SET current (ISD) versus gate voltagesVG1,VG2, at an applied bias ofVSD=0.5 mV, showing breaks inISDdue to charging of D2. (g)VG1projections ofISD, corresponding to the solid and dashed lines inf. The shift of the SET bias point due to charging of D2and the current contrast due to charge sensing are indicated by ΔVG1and ΔI, respectively. Figure 1: Spin readout architecture for donor clusters. ( a ) Central part of the device (in yellow), patterned by desorbing the hydrogen mask (in blue), showing the SET island (D 1 ), the few-donor quantum dot (D 2 ), and the innermost sections of the source and the drain leads of the SET. Spin-dependent tunnelling between D 1 and D 2 is shown schematically. ( b ) The overall device, showing the layout of the two gates (G 1 , G 2 ) and the extensions of the S and D leads. The white box shows the area shown in a . ( c ) Close-up image of D 2 , overlaid by a grid with dimer-row spacing, revealing the exposed silicon dimers. ( d , e ) Schematic representation of D 2 , showing sites suitable for P donor incorporation in green and the rest in yellow. The set of four white circles show two possible configurations of the P donors. ( f ) Map of SET current ( I SD ) versus gate voltages V G1 , V G2 , at an applied bias of V SD =0.5 mV, showing breaks in I SD due to charging of D 2 . ( g ) V G1 projections of I SD , corresponding to the solid and dashed lines in f . The shift of the SET bias point due to charging of D 2 and the current contrast due to charge sensing are indicated by Δ V G1 and Δ I , respectively. Full size image The lithographic template of D 2 ( Fig. 1c ) reveals two rows of five adjacent Si dimers (outlined with green ellipses in Fig. 1d ), which can accommodate a maximum of four P donors (see Supplementary Fig. S1 and Supplementary Methods ) [11] . Two possible configurations of these four donors are shown by the white circles. Being closely packed within an area of 1.5 nm × 2 nm, the largest possible separation between the donors is ≈2 nm ( Fig. 1d ), which is smaller than the Bohr radius of a single P donor in Si ( a B =2.5 nm). Therefore, the donor cluster D 2 behaves as a single quantum dot. D 2 is tunnel coupled to D 1 , so that charging and discharging of D 2 occur by exchanging electrons with D 1 , eliminating the need for any additional electron reservoir. Change in the charge state of D 2 results in a drastic change of the SET conductance. This is revealed in Fig. 1f , where the SET current is mapped as a function of V G1 and V G2 for a fixed source–drain bias ( V SD =0.5 mV). Each line corresponds to charge transitions of D 1 and exhibits discrete breaks, which reflects a shift of the SET bias point in capacitive response to charging and discharging of D 2 . Three such lines of breaks, denoted by A, B and C in Fig. 1f , correspond to three charge transitions of D 2 . A total of seven charge transitions could be identified for D 2 in a larger-area stability map [10] , but we saw no evidence of completely depleting the donor cluster within our available gate space. To quantify the sensitivity of charge detection, Fig. 1g shows V G1 projections of the stability map of Fig. 1f , for two different fixed values of V G2 (dotted and solid vertical lines in Fig. 1f ). These were chosen from either side of a particular charge transition line of D 2 (denoted by B) and have been superimposed on each other. The shift in the SET peak position (Δ V G1 =28 meV) due to charging of D 2 is large enough for the SET current to switch from its maximum to almost its minimum value (Δ I ), revealing nearly 100% contrast in charge sensing. This is an inherent advantage of charge sensing with a SET sensor, which enables high-fidelity spin readout [6] , [12] . Single-shot spin readout Having established the suitability of a STM-patterned SET for high contrast charge sensing [10] , we now demonstrate single-shot spin readout in this architecture, following the protocol initially developed by Elzerman et al . [13] This technique depends on spin-to-charge conversion by application of a magnetic field ( B ) and tracking in real time the current response of the SET to a three-level gate voltage pulse which loads, reads, and empties the up (|↑ >) and down (|↓>) spin states of D 2 ( and , respectively). We apply a three-level gate voltage pulse at the transition point shown in Fig. 2a (line B in Fig. 1f ), with the blue, brown and orange points representing the load, read, and empty positions, respectively. In the load phase, both and are pulled below μ D1 , whereby an electron of either spin-state tunnels onto D 2 , after a characteristic tunnelling time, τ load . This switches the SET ‘off’ and is seen in the single-shot current response as a sudden drop of I SD to its minimum value (see load columns in Fig. 2a ). 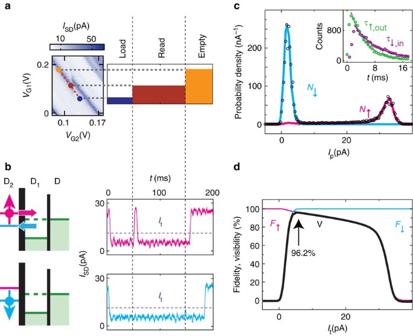Figure 2: High-fidelity single-shot spin readout. (a) A section of the stability plot of the SET and the applied three-level gate voltage pulse for single-shot spin readout. (b) Spin-dependent SET current response, showing a current peak for |↑> (top) and no peak for |↓> (bottom) detection. (c) Histogram of the current response maxima (Ip) for a fixed time interval (Δt=40 ms) in the readout phase, revealing two well-separated peaks. This distribution is fitted with the sum of two calculated histogramsN↑(pink) andN↓(blue). Inset: histogram of the tunnel-out times of the |↑> (green) and subsequent tunnel-in times of the |↓> (purple) electrons. Exponential fits to the histograms provide the corresponding tunnel rates, necessary for calculation ofN↑andN↓. (d) Readout fidelities (F↑andF↓) and visibility (V) as a function of threshold current,It. In the read phase, the pulse amplitude is so chosen that Figure 2: High-fidelity single-shot spin readout. ( a ) A section of the stability plot of the SET and the applied three-level gate voltage pulse for single-shot spin readout. ( b ) Spin-dependent SET current response, showing a current peak for |↑> (top) and no peak for |↓> (bottom) detection. ( c ) Histogram of the current response maxima ( I p ) for a fixed time interval (Δ t =40 ms) in the readout phase, revealing two well-separated peaks. This distribution is fitted with the sum of two calculated histograms N ↑ (pink) and N ↓ (blue). Inset: histogram of the tunnel-out times of the |↑> (green) and subsequent tunnel-in times of the |↓> (purple) electrons. Exponential fits to the histograms provide the corresponding tunnel rates, necessary for calculation of N ↑ and N ↓ . ( d ) Readout fidelities ( F ↑ and F ↓ ) and visibility ( V ) as a function of threshold current, I t . Full size image This is shown in the schematic illustrations of Fig. 2b . Here, I SD remains a minimum if a |↓> electron is loaded (see read column of lower panel in Fig. 2b ). On the other hand, if an |↑> electron is loaded, it tunnels back to D 1 and subsequently, a |↓> electron loads onto D 2 . This results in a peak in the SET current response (read column of upper panel in Fig. 2b ), as the SET is switched ‘on’ for a short while. In the final empty phase, D 2 is unloaded regardless of the spin state by plunging both and above μ D1 . This switches the SET ‘on’, until the next load phase starts. An isolated spike of the SET current in the read phase thus serves as an evidence of a |↑> electron being detected in this single-shot electrical spin readout scheme. For quantum computing applications, it is important to assess the fidelity of this detection process, that is, the probability of identifying the electronic spin state correctly from the current response of the SET. To quantify spin readout fidelity, we investigate the peak values of the SET current ( I p ), recorded over a certain time interval Δ t =40 ms in the read phase, for 20,000 traces. The distribution of I p is shown by the open circles in Fig. 2c , where the peak at high (low) I p is consistent with the current response of the SET for detection of the |↑> (|↓>) state. This distribution represents the sum , where N ↑ and N ↓ are the separate histograms for each spin configuration. N ↑(↓) cannot be deduced experimentally, but can be obtained by numerical modelling [6] , knowing the peak height (Δ I ), the detection bandwidth (300 Hz) and characteristic times for |↑>–(|↓>) electron tunnelling out of (onto) D 2 , τ ↑,out ( τ ↓,in ). Values of τ ↑,out =3.9 ms and τ ↓,in =6.9 ms were obtained from exponential fits to the histograms of the peak position and width, respectively, as shown in the inset of Fig. 2c . The calculated histograms for N ↑ (pink) and N ↓ (blue) sum up to match very well with the recorded distribution of I p in Fig. 2c . From the N ↑(↓) histograms, the readout fidelities of the |↑> and |↓> spin states, F ↑ and F ↓ , as well as the readout visibility, defined as V = F ↓ + F ↑ −1, can be determined as a function of threshold current I t and are shown in Fig. 2d . As evident in the plot, the visibility reaches a maximum of V =96.2% at an optimum threshold current of I t =5.4 pA, where F ↑ =96.4% and F ↓ =99.8%. However, a more rigorous estimate of visibility, taking spin-to-charge conversion losses into account, leads to V =93.4% (details in Supplementary Fig. S2 and Supplementary Note 1 ). Determining T 1 in P-donor clusters Having established the feasibility of discriminating the spin states with sufficiently high fidelity, we now turn to measurement of T 1 . To determine T 1 , single-shot current response of the SET is monitored for varying lengths of the load pulse t load . As t load is made longer, the fraction of |↑> detected in the readout phase decays exponentially, due to relaxation to the ground |↓> state. 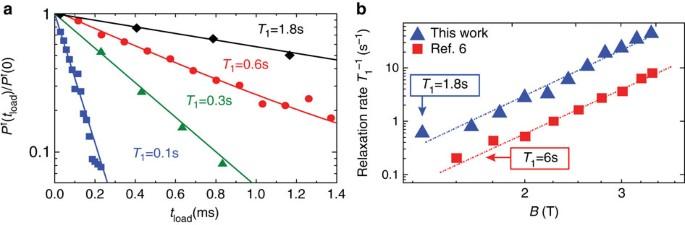Figure 3: Spin-lattice relaxation time of a P donor cluster. (a) Normalized |↑> fraction as a function oftload, for differentB-fields from 1.2 T (black diamonds) in steps of 0.4–2.6 T (blue squares). Exponential fit to the data yieldsT1. (b)B-field dependence ofof the device, together with that of an implanted donor (data from ref.6). Figure 3a shows this decay of the |↑> fraction at different magnetic fields. An exponential fit to the data yields T 1 , which for B =1.2 T is ≈1.8 s. Plotting the decay rates at different magnetic fields, we find a B 5 dependence of , as shown by the blue triangles in Fig. 3b . For comparison, we plot in the same figure, similar data for a single implanted P donor (reproduced from ref. 6 ), wherein the spin-lattice relaxation time was found to follow , with K 5 =0.015 T −1 s −1 . The B 5 dependence of reflects spin relaxation via the acoustic-phonon-mediated valley repopulation mechanism [14] , at the limit (ref. 6 ). Our data therefore strongly suggest that the same mechanism as for the case of single P donors in Si is also responsible for relaxation of the many-electron spin excited state, hosted by the P-donor cluster. Figure 3: Spin-lattice relaxation time of a P donor cluster. ( a ) Normalized |↑> fraction as a function of t load , for different B -fields from 1.2 T (black diamonds) in steps of 0.4–2.6 T (blue squares). Exponential fit to the data yields T 1 . ( b ) B -field dependence of of the device, together with that of an implanted donor (data from ref. 6 ). Full size image Single-shot spin readout was also attempted at a few other triple points. For other transitions along line B (same charge state of D 2 ), we measured similar values of T 1 . However, spin readout could not be performed for transitions on line A (line C), which represents one electron less (more) on D 2 , which is consistent with pairwise spin filling. Further insight on the absolute values of T 1 can be obtained by analysing the coefficient K 5 , which is an order of magnitude higher ( K 5 =0.134T −1 s −1 ) in our case. All parameters in K 5 are related to the the silicon bulk [6] , [14] except for the valley–orbit splitting (Δ E V ), which is sensitive to the nature of confinement potential, and hence to the number and distribution of the P donors defining the quantum dot. K 5 scales , which suggests that for the P-donor cluster Δ E V ≈3.5 meV. Interestingly, a very similar valley–orbit splitting has been observed for an exciton bound to a P in Si (ref. 15 ). Although an exact estimate of the valley–orbit splitting is computationally expensive for the system studied here, the lower value observed (compared with single P donors ( =10.6±0.2 meV (ref. 16 )) can be attributed to screening and correlation effects in a multi-electron quantum dot. A larger Δ E V , and hence a longer T 1 , will therefore be expected for the spin excited state of the last electron bound to the same quantum dot. Donor clusters as hosts for single-spin qubits The above results indicate that a long spin-lattice relaxation time can be retained even when single electronic spins are confined to small P-donor clusters. This fact opens up the prospect of using donor clusters as hosts for single-spin qubits and can be of significant consequence in performing single qubit rotations in a large array of Si:P qubits, as required for a practical quantum computing architecture. A daunting challenge of performing single qubit rotations with qubit arrays hosted by individual P donors is to excite electron spin resonance (ESR) transitions of a particular qubit, without affecting neighbouring ones. To achieve this selectivity, tuning ESR transitions of a targeted qubit into resonance with a globally applied microwave field (typically 30–40 GHz), by electrical control of the hyperfine coupling between the electron- and the donor-nuclear spins, has been proposed [17] . The ESR frequency of a single-P-donor qubit in a static magnetic field B is given by where h is the Planck’s constant; μ n = e /2 m n , the nuclear magneton; g n , the nuclear gyromagnetic ratio; and A ( E ) and g e ( E ), the electric field ( E ) tunable hyperfine coupling and electron gyromagnetic ratio, respectively. Here, we have included the E -field dependence of the g factor, which was ignored in previous donor spin qubit proposals [17] , but was measured in ESR experiments [18] . The selectivity of single qubit rotation in the canonical scheme relies on Stark shift of A ( E ) only to bring v in resonance with the microwave field ( v MW ), while all others qubits stay sufficiently detuned. However, the Stark tunability of A ( E ) (≈0.4 MHz/(MV/m) 2 ) and of the spin–orbit interaction μ B g e ( E ) (≈0.3 MHz/(T(MV/m) 2 )) may be insufficient to achieve the frequency shifts necessary for a required single qubit rotation fidelity (>10 −5 ) in realistic E -fields (≤10 MV m −1 ). On the basis of atomistic tight-binding modelling, in this section, we discuss that by hosting consecutive single-spin qubits in an array of clusters with different number of P donors, a ‘built-in’ selectivity of ESR frequencies can be achieved naturally. This arises due to the extreme sensitivity of the hyperfine coupling to the number and distribution of nuclear spins (see Supplementary Fig. S3 ). To demonstrate this, we plot in Fig. 4a the E -field (applied along the [1 0] direction) dependence of the ESR transition frequencies of both a single-donor (red lines) and a 2-P-donor cluster (blue lines), in a static magnetic field B =1.5 T. Such a two donor cluster (shown in the inset) can be realised by STM patterning (see Methods). 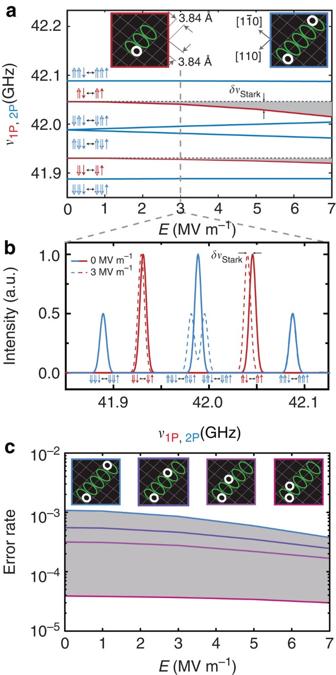Figure 4: ESR addressability of 1-P and 2-P qubits. (a)E-field (applied along [10]) dependence of ESR transition frequencies (blue lines) atB=1.5 T of the 2-P cluster (patterned along [110]), shown in the right panel of the inset. The same data for a single P donor (shown in the left panel of the inset) are shown by the red lines. (b) A schematic spectral representation of calculated resonance frequencies for 1-P and 2-P cluster atE=0 (solid) andE=3 MV m−1(dashed) using a peak width of ≈8 MHz (ref.9). (c)E-field dependence of the error rate, that is, the probability of exciting an ESR transition of the 2-P qubit (1-P qubit), when the global microwave field is in resonance with a transition of the 1-P qubit (2-P qubit), for different inter-donor separations (as shown in the inset). The oscillating magnetic field,Bac=10−4T, and the frequency difference correspond to thetransition of the 1-P qubit and thetransition of the 2-P qubit (see main text). The four blue lines in the plot correspond to the four possible ESR transitions between the eight eigenstates of the three-spin (one electron and two P nuclei) system, obtained by solving the effective spin Hamiltonian Figure 4: ESR addressability of 1-P and 2-P qubits. ( a ) E -field (applied along [1 0]) dependence of ESR transition frequencies (blue lines) at B =1.5 T of the 2-P cluster (patterned along [110]), shown in the right panel of the inset. The same data for a single P donor (shown in the left panel of the inset) are shown by the red lines. ( b ) A schematic spectral representation of calculated resonance frequencies for 1-P and 2-P cluster at E =0 (solid) and E =3 MV m −1 (dashed) using a peak width of ≈8 MHz (ref. 9 ). ( c ) E -field dependence of the error rate, that is, the probability of exciting an ESR transition of the 2-P qubit (1-P qubit), when the global microwave field is in resonance with a transition of the 1-P qubit (2-P qubit), for different inter-donor separations (as shown in the inset). The oscillating magnetic field, B ac =10 −4 T, and the frequency difference correspond to the transition of the 1-P qubit and the transition of the 2-P qubit (see main text). Full size image where s (σ z ) is the Pauli (−Z) matrix, with z representing the direction of the B -field, and e and n, i referring to the electron and the two P nuclei, respectively. The strength of the hyperfine coupling between the electron and the two P nuclear spins ( A i ( E )) (ref. 19 ), as well as the electronic g factor ( g e ( E )) (ref. 20 ), has been calculated within the tight-binding formalism (see Methods). We found that the Stark shift of the g factor is at least an order of magnitude weaker for the 2-P cluster than for 1-P (see Supplementary Note 2 ). The E -field dependence of the ESR transition frequencies corresponding to the single-P-donor qubit is also shown in the same plot. At E =0, the smallest difference in the ESR frequencies of the 1-P and the 2-P qubits, is ≈40 MHz. For the entire range of the studied E -field, δν is significantly larger than the Stark shift of ESR frequencies of a single P donor ( δν Stark in Fig. 4a ). Comparison between δν and δν Stark is illustrated in Fig. 4b , which schematically plots ESR transitions for a single P and a 2-P cluster at E= 0 and 3 MV m −1 , the latter representing an E -field where a bulk P donor is likely to ionize [21] . On the basis of the values of δv , we can estimate the error rates from the Rabi solution: where and B ac is the strength of the oscillating magnetic field due to the global microwave field. Assuming B ac =10 −4 T, the single qubit rotation operation time for the targeted qubit, t =1/(4 γ | δν =0 )=90 ns. The error rate, that is, the probability of rotating the untargeted qubit (for the smallest δν , as defined above) is given by the prefactor of equation (5), and is P ≈10 −3 . We note that this value of P is the most conservative estimate of the error rate. First, we have considered an inter-donor separation, which is the largest possible in a STM pattern of five dimers. For smaller inter-donor separations, the error rate can be suppressed further. This is shown in Fig. 4c for other 2-donor configurations. Second, we have assumed that for both 1-P and 2-P qubits, the nuclear spins are initialized in their respective ground states ( and ), which is the nuclear configuration where the electron resonance frequencies are the closest. If instead the 1-P qubit was initialized in the state, then P can be as small as 10 −5 , as MHz. We note that the expected nuclear spin relaxation time ( T ln ≈hours at 100 mK) (ref. 22 ) means that this nuclear configuration can be maintained for extremely long times. Therefore, hosting alternate spin qubits in 1-P and 2-P donors provides a viable route to perform high-fidelity single-qubit rotation in a globally applied microwave field. A remaining challenge, however, for this proposal is the experimental demonstration of single-donor placement within clusters with atomic precision accuracy, allowing the lowest error rates. To date the highest accuracy that has been achieved is ±1 lattice spacing [23] , and work is currently underway to increase this. In summary, we have demonstrated high-fidelity projective spin readout in a multi-P donor cluster, patterned in an atomically precise charge-sensing architecture. Importantly, we show long relaxation times (≈seconds), comparable to that of a single P donor in silicon. Using tight-binding calculations to determine the difference in hyperfine coupling in donor clusters of different sizes, we demonstrate the applicability of these systems for qubit addressability in a globally applied magnetic field. Device fabrication The device was fabricated on the (2 × 1) reconstructed surface of a n-doped (1–10 Ωcm) Si(001) wafer, in an ultra-high-vacuum STM chamber. After removal of the native oxide, the surface was first passivated with a monolayer hydrogen mask, and then patterned with the STM tip (4–7 V, 5–10 nA) to create the device template ( Fig. 1a ). Subsequent exposure to PH 3 gas and annealing at 350 °C for 1 min led to P incorporation, selectively within the device template. Once realized, the whole device was overgrown with ≈25-nm epitaxial Si in the same chamber. Aluminium leads were then fabricated ex situ by standard electron beam lithography and metallization techniques, to make Ohmic contacts to the buried device. Surface chemistry of P incorporation Within the lithographic pattern of D 2 ( Fig. 1c–e ), only the two rows of five Si dimers (marked by green ellipses) can incorporate P donors, while the rest (in yellow) cannot. This is understood by considering the series of dissociative surface chemical processes, which leads to P incorporation in silicon from the gaseous PH 3 precursor [11] . The schematics of Supplementary Fig. S3 illustrate these processes. Dosing at sufficiently high rate leads to dissociation of PH 3 molecules into PH 2 +H, at every exposed Si dimer site ( Supplementary Fig. S3a ). This inhibits any further reaction at room temperature. However, when the surface is subsequently heated up to 350 °C for annealing, one PH 2 fragment recombines with a H atom and desorbs as PH 3 ( Supplementary Fig. S3b ). This results in one dimer site being available for immediate dissociation of another PH 2 to PH+H ( Supplementary Fig. S3c ). Finally, the third PH 2 desorbs as well, making room for further dissociation of the PH to P+H ( Supplementary Fig. S3d ). Still under annealing conditions, the P atom exchanges site with a Si atom of the top layer, thereby being incorporated ( Supplementary Fig. S3e ). As evident from the schematic diagrams, five bare-silicon sites (or 2.5 adjacent Si dimers) are required to incorporate a P donor. This is only satisfied within the two rows of five Si dimers in Fig. 1c–e , and makes the most likely donor count of D 2 to be four. On the basis of the understanding of the dissociative surface chemical processes, it is also evident that the five dimer patches of Fig. 4 can host a maximum of two P donors. Electrical measurements For all electrical measurements, the device was mounted on a high-frequency printed circuit board within a copper enclosure, thermally anchored to the cold finger of a dilution refrigerator, with a base temperature of ≈100 mK. Direct current voltage was applied to the two gates and added to the voltage pulses generated by an arbitrary waveform generator. The SET current, I SD , was amplified, converted into a voltage signal at room temperature, filtered with an 8th order low-pass Bessel filter, and measured with a fast digitizing oscilloscope. Calculation of hyperfine coupling The strength of hyperfine coupling, A , is proportional to the probability density of the electron wavefunction at the site of the donor atom r i (ref. 19 ). An applied electric field ( E ) distorts the wavefunction and, therefore, modifies A . To calculate the E dependence of A , the electron wavefunctions were first obtained from the semi-empirical tight-binding method in the Nanoelectronic Modeling tool (NEMO-3D), as described in ref. 19 . In addition to the contact hyperfine components A , we also calculate the anisotropic components of the full hyperfine tensor B (as described in ref. 24 ) to estimate whether the modified wavefunction of an electron bound to a donor cluster poses an obstacle to the coherent manipulation of the electron spin. We found for the 2-P cluster depicted in Fig. 4a kHz, kHz, kHz, all approximately 0.001 times the contact hyperfine term. The tight-binding method is an atomistic full band method that effectively captures the multi-valley structure and valley–orbit interactions present in silicon, providing a highly accurate description of Stark-shifted single-donor states. The method has been very effective in explaining a variety of donor experiments in silicon [23] , [25] . How to cite this article: Büch, H. et al . Spin readout and addressability of phosphorus-donor clusters in silicon. Nat. Commun. 4:2017 doi: 10.1038/ncomms3017 (2013).